Limitations on quantum key repeaters A major application of quantum communication is the distribution of entangled particles for use in quantum key distribution. Owing to noise in the communication line, quantum key distribution is, in practice, limited to a distance of a few hundred kilometres, and can only be extended to longer distances by use of a quantum repeater, a device that performs entanglement distillation and quantum teleportation. The existence of noisy entangled states that are undistillable but nevertheless useful for quantum key distribution raises the question of the feasibility of a quantum key repeater, which would work beyond the limits of entanglement distillation, hence possibly tolerating higher noise levels than existing protocols. Here we exhibit fundamental limits on such a device in the form of bounds on the rate at which it may extract secure key. As a consequence, we give examples of states suitable for quantum key distribution but unsuitable for the most general quantum key repeater protocol. When a signal is passed from a sender to a receiver, it inevitably degrades due to the noise present in any realistic communication channel, for example, a cable or free space. The degradation of the signal is typically exponential in the length of the communication line. When the signal is classical, degradation can be counteracted by the use of an amplifier that measures the degraded signal and, depending on a threshold, replaces it by a stronger signal. When the signal is quantum mechanical (for example, encoded in non-orthogonal polarizations of a single photon), such an amplifier cannot work anymore, since the measurement inevitably disturbs the signal [1] , and, more generally, since quantum mechanical signals cannot be cloned [2] . Sending a quantum signal, however, is the basis of quantum key distribution (QKD), a method to distribute a cryptographic key, which can later be used for perfectly secure communication between sender and receiver [3] . The degradation of sent quantum signals therefore seems to place a fundamental limit on the distance at which secure communication is possible thereby severely limiting its applicability in the internet [4] , [5] , [6] . A way around this limitation is the use of entanglement-based QKD schemes [7] , [8] in conjunction with a so-called quantum repeater [9] , [10] . This amounts to distributing n Einstein–Podolsky–Rosen (EPR) pairs between Alice and Charlie (an untrusted telecom provider) and between Bob and Charlie. Imperfections due to noise in the transmission are compensated by distillation, yielding ≈ E D × n perfect EPR pairs. Here E D denotes the distillable entanglement of the imperfect EPR pair, that is, the optimal rate at which perfect EPR pairs can be distilled from imperfect ones. The EPR pairs between Charlie and Bob are then used to teleport the state of Charlie’s other particles to Bob. This process, known as entanglement swapping, results in EPR pairs between Alice and Bob [11] (see Fig. 1 ). When Alice and Bob make appropriate measurements on these EPR pairs, they obtain a sequence of secret key bits, that is, an identical but random sequence of bits that is uncorrelated with the rest of the universe (including Charlie’s systems), enabling secure communication. The described scheme with one intermediate station effectively doubles the distance over which QKD can be carried out. This abstract view of the quantum repeater will be sufficient for our purpose. The full proposal of a quantum repeater in fact allows to efficiently extend the distance arbitrarily even if the local operations are subject to a limited amount of noise [9] . The implementation of quantum repeaters is therefore one of the focal points of experimental quantum information science [10] . 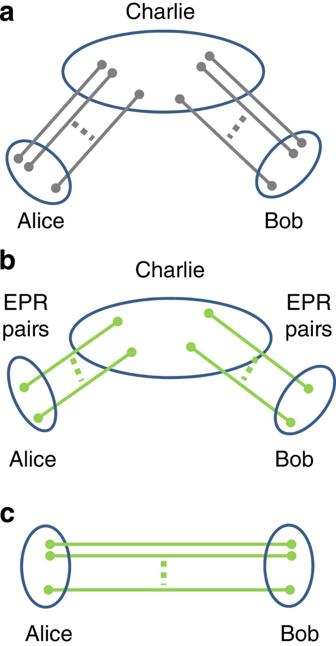Figure 1: Quantum repeater. (a) Alice and Charlie—and similarly Charlie and Bob—distil EPR pairs from noisy states (grey). (b) Charlie uses the EPR pairs (green) he shares with Bob to teleport his part of the states he shares with Alice to Bob. (c) Alice and Bob share EPR pairs. Figure 1: Quantum repeater. ( a ) Alice and Charlie—and similarly Charlie and Bob—distil EPR pairs from noisy states (grey). ( b ) Charlie uses the EPR pairs (green) he shares with Bob to teleport his part of the states he shares with Alice to Bob. ( c ) Alice and Bob share EPR pairs. Full size image Owing to the tight connection between the distillation of EPR pairs and QKD [12] , [13] , it came as a surprise that there are bound entangled states (that is, entangled states with vanishing distillable entanglement) from which the secret key can be obtained [14] . With the help of a quantum repeater as described above, however, the secret key contained in such states cannot be extended to larger distances, as the states do not allow for the distillation of EPR pairs. This raises the question of whether there may be other ways to extend the secret key to arbitrary distances than by entanglement distillation and swapping, other quantum key repeaters. In this work, we introduce and formally define the concept of a quantum key repeater. We then study the associated quantum key repeater rate. It is always at least as large as the rate that can be obtained in a quantum repeater protocol and we raise the question whether it could be larger (and in particular non-zero for bound entangled states). Our main results consist of upper bounds on this quantity which we use to show that there are quantum states with extreme behaviour—state with a large key rate but with a negligible quantum key repeater rate. We thus demonstrate the fundamental limitations on quantum key repeaters. The quantum key repeater rate We analyse the quantum key repeater rate K A↔C↔B at which a protocol—only using local operations and classical communication (LOCC)—is able to extract private bits between Alice and Bob from entangled states, which each of them shares with Charlie (see Fig. 2 ). See Supplementary Note 1 for a formal definition of the key repeater rate. By a private bit, we mean an entangled state containing a unit of privacy paralleling the EPR pair as a unit of entanglement [14] , [15] . 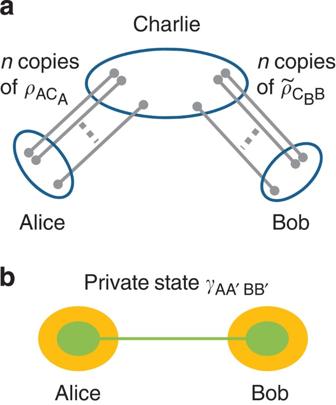Figure 2: Quantum key repeater. (a) Multiple copies of noisy statesρand, shared by Alice and Charlie and by Charlie and Bob, respectively, are transformed by means of LOCC into (b) a private stateγ(green-yellow) between Alice and Bob. Mathematically, private bits are entangled states of the form Figure 2: Quantum key repeater. ( a ) Multiple copies of noisy states ρ and , shared by Alice and Charlie and by Charlie and Bob, respectively, are transformed by means of LOCC into ( b ) a private state γ (green-yellow) between Alice and Bob. Full size image where A and B are qubits that contain the key bits, corresponding to the rows and columns in the matrix. The AB subsystem is called the key part. A′ and B′ are each a d -dimensional systems, forming the so-called shield part. X is a d 2 -by- d 2 matrix with || X || 1 =1 (see also Fig. 3 ). γ AA′BB′ can also be presented in the form , where σ A′B′ is some state, and , where U 0 and U 1 are unitaries acting on σ A′B′ . This operation is called twisting. It is now easy to see that the bit that Alice and Bob obtain when they measure A and B in the computation basis is a key bit, that is, it is random and secure, that is product with a purification of γ held by the eavesdropper. The relation between X and σ A′B′ is given by . 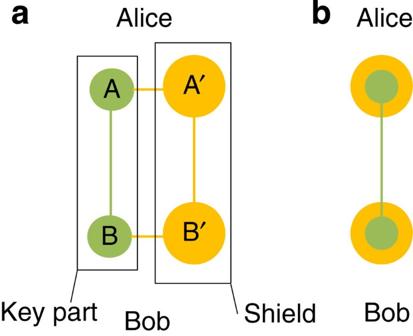Figure 3: The private stateγAA′BB′. (a) Bipartite state with four subsystems A, A′, B and B′. The subsystems AB form the ‘key part’ (green) which, due to the ‘shield part’ A′B′ (yellow), is secure against an eavesdropper. (b) Icon of a private bit. Figure 3: The private state γ AA′BB′ . ( a ) Bipartite state with four subsystems A, A′, B and B′. The subsystems AB form the ‘key part’ (green) which, due to the ‘shield part’ A′B′ (yellow), is secure against an eavesdropper. ( b ) Icon of a private bit. Full size image Note that just as the definition of the distillable key [14] , [16] , the definition of the quantum key repeater rate is information-theoretic in nature. The role of Charlie here merits special attention. While he participates in the LOCC protocol like Alice and Bob do, he is not a ‘trusted party’; indeed, at the end of the protocol, Alice and Bob wish to obtain private bits, whose privacy is not compromised even if at that point Charlie passes all his remaining information to the eavesdropper. We also note that well-known techniques from quantum information theory [17] , [18] allow to conclude that the obtained rate of private bits can be made unconditionally secure [19] , [20] , [21] . In the following, we will describe our main results, which demonstrate that the performance of quantum key repeaters beyond the use of entanglement distillation is severely limited. Some private states cannot be swapped Our first result takes as its starting point the observation that there are private bits that are almost indistinguishable from separable states by LOCC [22] . To see this, consider the state which is obtained from γ , when Alice and Bob measure the key part of their state in the computational basis. An example is given by the choice , where the u ij are the entries in the quantum Fourier transform in dimension d . For this choice of X , is separable. The distinguishability under LOCC operations is measured in the norm , which is bounded by the distinguishability under global maps preserving the positivity under the partial transpose (ref. 23 ). This can further be bounded by , which is easily calculated as . Γ indicates the partial transpose, that is, the transpose of one of the systems [24] . Suppose now that a quantum repeater protocol applied to two copies of the latter state, shared by Alice and Charlie and Bob and Charlie, respectively, successfully outputs a private bit between Alice and Bob. This could be regarded as the privacy analogue to entanglement swapping. Then, if Alice and Bob joined their labs, they could distinguish this resulting state from a separable state, as separable states are well distinguishable from private states by a global measurement [14] . This implies an LOCC procedure for Alice and Bob (jointly) and Charlie to distinguish the initial private bits γ ⊗ γ from separable states: first run the quantum key repeater protocol and then perform the measurement. This, however, is in contradiction to the property that the private state γ (and hence γ ⊗ γ ) is almost indistinguishable from separable states under LOCC. In conclusion, this shows that such private bits cannot be successfully extended to a private bit between Alice and Bob by any LOCC protocol acting on single copies (see Supplementary Note 2 ). Bounding the quantum key repeater rate Although intuitive, the above argument only bounds the repeated key obtained from a single copy of input states. The language of entanglement measures allows us to formulate this argument asymptotically as a rigorous distinguishability bound on the rate K A↔C↔B for general states ρ and : where the right-hand side is the regularized LOCC-restricted relative entropy distance to the closest separable state [25] : , where D C↔AB ( ρ )=inf σ sup M D ( M ( ρ )|| M ( σ )) with the minimization over separable states σ , the maximization over measurements implementable by LOCC with respect to the C:AB partition and D the relative entropy distance. The proof is given in Supplementary Note 3 . Arguably, it is difficult, if not impossible, to compute this expression. But noting that this bound is invariant under partial transposition of the C system, we can easily upper bound the quantity for all known bound entangled states (these are the ones with positive partial transpose) in terms of the regularised relative entropy of entanglement of the partially transposed state . The relative entropy of entanglement is given by E R ( ρ )=min σ D ( ρ || σ ) where the minimization extends over separable states; the regularization is analogous to the one above. If we restrict to forward communication from Charlie and , the squashed entanglement measure provides a bound: . The squashed entanglement is given as (one half times) the minimal conditional mutual information when minimizing over all extensions of the state (we condition on the extending system). Using invariance under partial transposition directly on the hypothetical quantum key repeater protocol, we obtain for PPT states ρ and : where K D is the key rate, that is, the rate at which secret key can be extracted from ρ by LOCC. The same holds for . The proof can be found in Supplementary Note 4 . We will now give an example of a state for which the key rate is large, but the bounds and hence the quantum key repeater rate, are arbitrarily small. Guided by our intuition, we would like to consider the private bit γ from above whose partial transpose is close to a separable state. The state, however, is not PPT, as no private bit can be PPT [14] . Fortunately, it turns into a PPT state ρ under mixing with a small amount of noise and we find K A↔C↔B ( ρ ⊗ ρ )≈0 while K D ( ρ )≈1. This leads us to the main conclusion of our paper—there exist entangled quantum states that are useful for QKD at small distances but that are virtually useless for long-distance QKD (see Fig. 4 ). 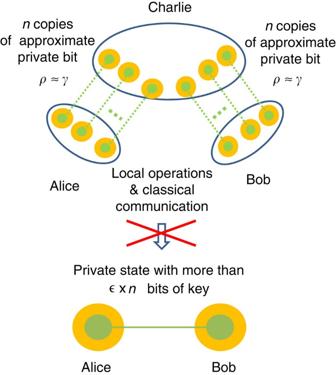Figure 4: Limitation on quantum key repeaters. Despite Alice and Charlie as well as Charlie and Bob sharing states containing almost n bits of secrecy there is no LOCC protocol between Alice, Charlie and Bob, which results in a non-negligible amount of secure key between Alice and Bob. Figure 4: Limitation on quantum key repeaters. Despite Alice and Charlie as well as Charlie and Bob sharing states containing almost n bits of secrecy there is no LOCC protocol between Alice, Charlie and Bob, which results in a non-negligible amount of secure key between Alice and Bob. Full size image Bounding the entanglement of the output Finally, we present a different type of bound on the quantum key repeater rate based on the direct analysis of the entanglement of a concrete output state of a quantum repeater protocol: where E C denotes the entanglement cost of the state, the rate of EPR states needed to create many copies of the state. This bound, unlike the ones presented above, applies to all quantum states. In particular, it applies to certain states invariant under partial transposition, which escape the techniques presented before. Note that in the case of PPT states, one may partially transpose the states appearing on the right-hand side since K A←C↔B is invariant under partial transposition. The proof of equation (5) is obtained by upper bounding the squashed entanglement of the output state of the protocol using a manipulation of entropies resulting in the right-hand side of equation (5). The squashed entanglement in turn upper bounds the distillable key of the output state (which upper bounds the left hand side) [26] . For a detailed proof see Supplementary Note 5 . There, we also exhibit a private bit with a significant drop in the repeater rate when compared with the key rate. We further investigate the tightness of the bound (5) and, based on a random construction, show that the left hand side cannot be replaced by the entanglement cost of the output state. The preceding results pose limitations on the entanglement of the output state of a quantum key repeater protocol. As such, they support the PPT-square conjecture: assume that Alice and Charlie share a PPT state and that Bob and Charlie share a PPT state; then the state of Alice and Bob, conditioned on any measurement by Charlie, is always separable [27] , [28] , [29] . Reaching even further, and consistent with our findings, we may speculate that perhaps the only ‘transitive’ entanglement in quantum states, that is, entanglement that survives a quantum key repeater, is the distillable entanglement. One may also wonder whether apart from equation (5) there are other inequalities between entanglement measures of the in- and output states. In the context of algebro-geometric measures, this question has been raised and relations for the concurrence have been found [30] , [31] . Our work focuses on operational entanglement measures. States from which more key than entanglement can be extracted have recently been demonstrated experimentally in a quantum optical set-up [32] . These are exactly the private states discussed in Supplementary Note 2 ( X is the SWAP operator) with shield dimension equal to two. As our results for these states only become effective for higher shield dimensions, we cannot conclude that the single-copy key repeater drops when compared with the key contained in these states. This may be overcome by stronger theoretical bounds or experimental progress, which increases the shield dimension; we expect both improvements to be achieved in the near future. With this paper, we initiate the study of long-distance quantum communication and cryptography beyond the use of entanglement distillation by the introduction of the concept of a quantum key repeater. Even though the reported results provide limitations rather than new possibilities, we hope that this work will lead to a rethinking of the currently used protocols resulting in procedures for long-distance quantum communication that are both more efficient and that can operate in noisier environments. In the following, we will give a simple example of such a rethinking: assume that Alice and Charlie share a private bit that is almost PPT and thus requires a large shield system (see Supplementary Note 6 ). The quantum repeater based on quantum teleportation would thus require Bob and Charlie to share a large amount of EPR pairs to teleport Charlie’s share of to Bob. Alice and Bob can then extract one bit of secret key by measuring the state. Inspired by the work of Smith and Yard [33] , we show in Supplementary Note 6 that a single EPR pair and a particular state , which is so noisy that it contains no (one-way) distillable entanglement, are sufficient to obtain a large quantum key repeater rate (using only one-way communication from Alice and Charlie to Bob). We thus showed that there are situations in which significant amounts of distillable entanglement may be replaced by (one-way) undistillable states. How to cite this article: Bäuml, S. et al . Limitations on quantum key repeaters. Nat. Commun. 6:6908 doi: 10.1038/ncomms7908 (2015).